Sulphur-impregnated flow cathode to enable high-energy-density lithium flow batteries Redox flow batteries are promising technologies for large-scale electricity storage, but have been suffering from low energy density and low volumetric capacity. Here we report a flow cathode that exploits highly concentrated sulphur-impregnated carbon composite, to achieve a catholyte volumetric capacity 294 Ah l −1 with long cycle life (>100 cycles), high columbic efficiency (>90%, 100 cycles) and high energy efficiency (>80%, 100 cycles). The demonstrated catholyte volumetric capacity is five times higher than the all-vanadium flow batteries (60 Ah l −1 ) and 3–6 times higher than the demonstrated lithium-polysulphide approaches (50–117 Ah l −1 ). Pseudo- in situ impedance and microscopy characterizations reveal superior electrochemical and morphological reversibility of the sulphur redox reactions. Our approach of exploiting sulphur-impregnated carbon composite in the flow cathode creates effective interfaces between the insulating sulphur and conductive carbon-percolating network and offers a promising direction to develop high-energy-density flow batteries. Energy storage system is a critical enabling factor for deploying unstable and intermittent renewable power sources, such as solar and wind power sources [1] , [2] , [3] , [4] , [5] , [6] . Redox flow batteries (RFBs) are promising technologies for large-scale electricity storage, owing to its design flexibility in decoupling power and energy capacity [7] , [8] , [9] , [10] . However, the RFBs have been suffering from low energy density and low volumetric capacity, which significantly decreases its competitiveness for both stationary and transportation applications [11] , [12] , [13] , [14] . Increasing the energy density and volumetric capacity of RFBs has been one of the major research efforts for RFBs and has motivated several new design concepts to date. Lu and Goodenough [15] , [16] have proposed a hybrid flow battery using an alkaline metal (for example, lithium metal) and aqueous redox-active species (for example, ferricyanide) as cathodes, separated by a glass ceramic membrane. This unique concept creates high cell voltage between the aqueous cathode and the most electronegative alkaline metal. However, the hybrid configuration using lithium metal limits the scalability of energy and power of the lithium-negative electrode [17] , which can be achieved in an all-vanadium flow battery. The authors demonstrated a lithium-ferricyanide flow battery that operates at ~3.40 V with a coulombic efficiency >97%. Inspired by this concept, several groups have proposed to replace the ferricyanide redox couple with aqueous FeCl 3 /FeCl 2 (ref. 18 ) or I – /I 3 – (ref. 19 ) or aqueous polysulphide [20] to increase the concentration of the catholyte while keeping the solid lithium-metal anode for large cell voltage. One major drawback of the lithium/aqueous configuration is the need for a crack-free glass ceramic membrane, which is expensive (LICGC USD $90 cm −2 ( http://www.oharacorp.com/ ) versus Celgard separators <USD $0.1 cm −2 ( http://www.celgard.com/ )) and highly resistive (low ionic conductivity 1.0 × 10 −4 S cm −1 versus 9 × 10 −3 S cm −1 for organic electrolytes [21] ). To increase the volumetric capacity of lithium flow batteries ( Fig. 1a ) and eliminate the need for a glass ceramic membrane, two major approaches were reported, as illustrated in Fig. 1b,c . First, Yang et al . [12] proposed the concept of using nonaqueous lithium polysulphide in the catholyte [12] , [22] (with a carbon fibre electrode current collector) and have demonstrated a catholyte volumetric capacity of 50 Ah l −1 (108 Wh l −1 , average cell voltage 2.2 V against lithium metal) [12] using 5.0 M polysulphide catholyte. Inspired by this work, Fan et al . [23] replaced the carbon fibre electrode current collector with a carbon-percolating conducting network as a flow current collector ( Fig. 1b ), demonstrating Li-polysulphide flow batteries with a catholyte volumetric capacity of 117 Ah l −1 (234 Wh l −1 , average cell voltage 2.0 V against lithium metal) [23] . In this approach, the solid sulphur phase was purposely avoided due to the extremely low solubility and insulating nature of the solid sulphur, which sacrifices the theoretical volumetric capacity. Second, Duduta et al . [13] proposed the concept of semi-solid Li-ion flow batteries utilizing solid intercalation materials in a carbon (Ketjen black (KB))-percolating conducting network ( Fig. 1c ). In this approach, the solid intercalation materials are mechanically mixed with the conducting additives and organic electrolytes to form a suspension, which can be circulated in the catholyte (for example, LiCoO 2 ) and anolyte (for example, Li 4 Ti 5 O 12 ) separated by a polymeric separator. Recently, researchers have employed a similar approach to develop a semi-solid LiFePO 4 flow cathode (19 Ah l −1 : 12.6 vol% LiFePO 4 , achieved capacity 160 mAh g −1 ) [24] , and aqueous semi-solid LiFePO 4 flow cathode (16 Ah l −1 : 10.0 vol% LiFePO 4 , achieved capacity 150 mAh g −1 ) [25] . While the mechanically mixed intercalation semi-solid approach effectively increases the volumetric capacity of the flow batteries, the poor contacts between the large/insulating intercalation particles and the carbon network in the flow cathode become critical challenges [13] . 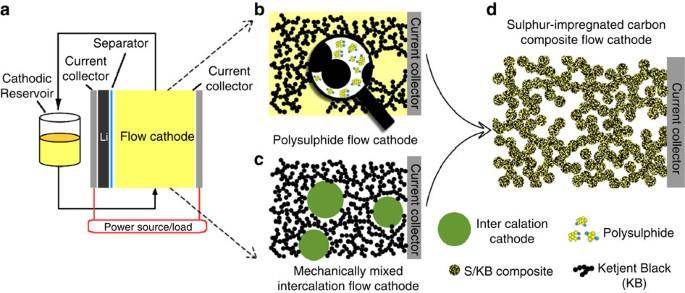Figure 1: Concept of a sulphur-impregnated carbon composite flow cathode. (a) Schematic representation of a nonaqueous lithium flow battery using (b) a polysulphide flow cathode12,22,23; (c) mechanically mixed intercalation flow cathode13,24; and (d) a new flow-cathode structure employing sulphur-impregnated Ketjen black composite suspended in the nonaqueous electrolyte described in this study. Figure 1: Concept of a sulphur-impregnated carbon composite flow cathode. ( a ) Schematic representation of a nonaqueous lithium flow battery using ( b ) a polysulphide flow cathode [12] , [22] , [23] ; ( c ) mechanically mixed intercalation flow cathode [13] , [24] ; and ( d ) a new flow-cathode structure employing sulphur-impregnated Ketjen black composite suspended in the nonaqueous electrolyte described in this study. Full size image In this work, we demonstrate a new flow-cathode concept that offers higher catholyte volumetric capacity compared with the above approaches, and alleviates contact issues between insulating active materials and the conductive carbon network. Our design employs sulphur-impregnated carbon (S/C) composite as a flow cathode ( Fig. 1d ) to achieve high-energy lithium-flow batteries with catholyte volumetric capacity ranging between 294 and 192 Ah l −1 at various current densities with long cycle life (>100 cycles), high columbic efficiency (90–94.5% at 100th cycle) and energy efficiency (82–83.7% at 100th cycle). The demonstrated catholyte volumetric capacity is >5 times higher than the state-of-the-art vanadium flow battery (60 Ah l −1 ) [3] , [26] and 3–6 times higher than the demonstrated Li-polysulphide approach (50–117 Ah l −1 ) [12] , [23] . Physical origins responsible for the enhanced volumetric capacity and superior electrochemical reversibility will be discussed. Design considerations of the S/C flow cathode The design of sulphur-impregnated carbon composite flow cathode offers three unique advantages compared with the existing approaches [12] , [13] , [23] , [24] , [27] . First, it exploits solid elemental sulphur (S 8 ) as the active material instead of polysulphide (Li 2 S 8 /Li 2 S 4 ) in the flow cathodes [12] , [23] . This increases the volumetric capacity of the flow cathode by 22.5% compared with polysulphide phase at a given S concentration. Previous studies [12] , [23] purposely avoided using solid sulphur due to its extremely low solubility and insulating nature. Here, we purposely go beyond the solubility limit of sulphur and exploit the solid phase to achieve high concentration of sulphur. Second, to address the concerns of insulating solid sulphur in the flow cathode, we impregnate sulphur with KB carbon rather than the conventional mechanical mixing approach reported for intercalation compounds [13] , [24] , [27] . We show that exploiting the sulphur-impregnated catholyte uniformly integrates the active materials (solid sulphur) and the conductive carbon-percolating network (KB), which enhances the utilization of insulating sulphur. The sulphur-impregnated carbon composite flow-cathode structure is inspired by well-established strategies for traditional solid sulphur electrodes [28] , [29] , [30] , [31] , [32] , [33] , [34] , [35] , [36] , [37] , [38] . Third, an unexpected advantage of using S/C composite is that the viscosity of the S/C composite catholyte is significantly lower than the mechanically mixed S+C catholyte (under the same S and carbon concentration, see Results). The reduced suspension viscosity significantly increases the maximum allowable concentration of sulphur in the catholyte, which boosts the theoretical volumetric capacity of the flow cathode. Table 1 compares the theoretical catholyte volumetric capacity of our approach with several reported nonaqueous flow cathodes (that is, the polysulphide flow cathode [12] , [23] and mechanically mixed intercalation cathode [13] , [24] ). All the volumetric percentages were calculated using the tap density for comparison (LiCoO 2 : 2.4 g cm −3 , LiFePO 4 : 0.78 g cm −3 , sulphur: 2.07 g cm −3 and KB: 0.12 g cm −3 ) (refs 24 , 39 , 40 , 41 ). The S/C composite catholyte concept offers higher volumetric capacity compared with the soluble polysulphide approach and the mechanically mixed intercalation approaches, owing to the increased active-material concentration and number of electrons transferred. Table 1 Theoretical volumetric capacity of flow cathodes. Full size table We examine the influences of (1) the mixing method of sulphur (mechanical mixing versus sulphur impregnation), (2) the concentration of carbon and (3) the concentration of sulphur on the electrochemical behaviour/performance of the S/C catholyte in Li-suspension cells (or ‘zero-gap’ cell, Supplementary Fig. 1 ). 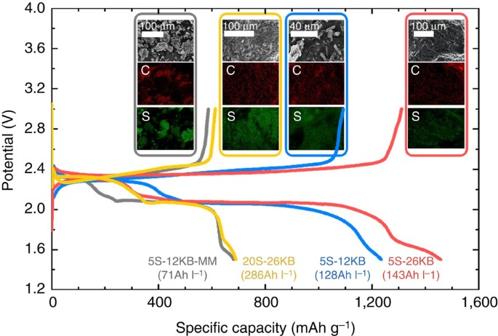Figure 2: Galvanostatic voltage profiles and SEM/EDX images. First galvanostatic discharge/charge profile of Li-suspension cells using sulphur–carbon catholytes of 5S–12KB-MM, 5S–12KB, 5S–26KB and 20S–26KB at C/9 (1C≡1,675 mA g−1). The electrochemical tests were replicated for more than three times. Insets: SEM/EDX images of pristine catholytes of 5S–12KB-MM, 5S–12KB, 5S–26KB and 20S–26KB. Figure 2 shows the first discharge/charge profiles and the scanning electron microscope/energy-dispersive X-ray spectroscopy (SEM/EDX) images of four sulphur–carbon catholytes including a mechanically mixed sulphur–carbon suspension with 5.0 vol% sulphur–12.0 vol% KB (that is, 5S–12KB-MM, 3.2 M [S]) and three sulphur-impregnated S/C composite suspensions (that is, 5.0 vol% sulphur–12.0 vol% KB (5S–12KB, 3.2 M [S]), 5.0 vol% sulphur–26.0 vol% KB (5S–26KB, 3.2 M [S]) and 20.0 vol% sulphur–26.0 vol% KB (20S–26KB, 12.9 M [S])). Figure 2: Galvanostatic voltage profiles and SEM/EDX images. First galvanostatic discharge/charge profile of Li-suspension cells using sulphur–carbon catholytes of 5S–12KB-MM, 5S–12KB, 5S–26KB and 20S–26KB at C/9 (1C≡1,675 mA g −1 ). The electrochemical tests were replicated for more than three times. Insets: SEM/EDX images of pristine catholytes of 5S–12KB-MM, 5S–12KB, 5S–26KB and 20S–26KB. Full size image High-energy catholyte enabled by sulphur impregnation Impregnation of sulphur with the conductive carbon matrix improves the electrical conductivity of the catholyte and enhances the interfacial contacts between the insulating solid sulphur and the carbon matrix, compared with a mechanically mixed suspension. The gravimetric discharge capacity of the mechanically mixed catholyte ( Fig. 2 , 5S–12KB-MM, 700 mAh g −1 ) is lower than that of the S/C composite catholyte ( Fig. 2 , 5S–12KB, 1,235 mAh g −1 ) by ~50%. This suggests that the utilization of sulphur in the catholyte is enhanced by the uniform intermixing of S and C using sulphur impregnation. The SEM/EDX image of the 5S–12KB catholyte shows that the S and C atoms are evenly distributed and overlapped across the composite suspension. On the other hand, the S and C atoms are separated in the mechanically mixed suspension (5S–12KB-MM). We employed the electrochemical impedance spectroscopy (EIS) technique to probe the influence of the sulphur-mixing method on the ohmic ( R ohm ), interfacial ( R int ) and charge-transfer resistances ( R ct ) of the S/C catholyte cells ( Fig. 3 ). 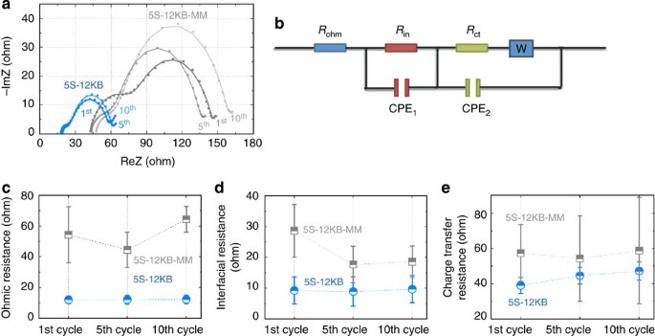Figure 3: EIS measurements of Li-suspension cells. (a) EIS data (dot symbols) and the fitting results (solid line) of 5S–12KB-MM and 5S–12KB Li-suspension cells after 1st, 5th and 10th discharge/charge cycles at C/9 (1C=1,675 mA g−1). (b) The equivalent circuit used to fit the EIS data shown ina. EIS-fitting results on (c) ohmic resistance, (d) interfacial resistance and (e) charge-transfer resistance for 5S–12KB-MM and 5S–12KB Li-suspension cells after 1st, 5th and 10th discharge/charge cycles. The EIS tests were replicated for three times. Figure 3a shows the EIS responses of 5S–12KB-MM and 5S–12KB after the 1st, 5th and 10th discharge/charge cycles with fitting results shown in Fig. 3c–e based on an equivalent circuit shown in Fig. 3b . Applying a well-recognized EIS physical model for Li–S/Li-ion batteries [23] , [42] , [43] , the high-frequency intercept has been attributed to the cell ohmic resistance, the middle-frequency semi-circle has been attributed to the interfacial resistance/capacitance of the catholyte and the low-frequency semi-circle has been attributed to the charge-transfer resistance/pseudocapacitance of the catholyte [23] , [42] , [43] . First, the S/C composite (5S–12KB) shows a threefold decrease in the ohmic resistance compared with the mechanically mixed sample ( Fig. 3c ), suggesting that the electrical conductivity of the catholyte network is improved with the well-intermixed S/C composite compared with the microscopically separated S+C mixtures. Second, the composite (5S–12KB) shows a 1.5–2-fold decrease in the interfacial resistance compared with the mechanically mixed sample ( Fig. 3d ). This can be attributed to the uniform intermixing of sulphur and carbon in the suspension, where small and accessible grains of sulphur are readily surrounded by the conductive KB. No significant difference can be concluded for the charge-transfer resistance ( Fig. 3e ) due to the large scattering of the mechanically mixed sample, which could be related to the inherent non-homogeneity of the mechanically mixed sample. Nevertheless, we show that impregnating insulating active materials with a conductive carbon matrix enhances the electrical conductivity and interfacial contacts of the catholyte, leading to the improved electrochemical performance of the catholyte. The subsequent cycles of the 5S–12KB and 5S–12KB-MM catholyte cells agree well with the observation in the first cycle discussed here ( Supplementary Fig. 2 ). Figure 3: EIS measurements of Li-suspension cells. ( a ) EIS data (dot symbols) and the fitting results (solid line) of 5S–12KB-MM and 5S–12KB Li-suspension cells after 1st, 5th and 10th discharge/charge cycles at C/9 (1C=1,675 mA g −1 ). ( b ) The equivalent circuit used to fit the EIS data shown in a . EIS-fitting results on ( c ) ohmic resistance, ( d ) interfacial resistance and ( e ) charge-transfer resistance for 5S–12KB-MM and 5S–12KB Li-suspension cells after 1st, 5th and 10th discharge/charge cycles. The EIS tests were replicated for three times. Full size image The viscosity of the flow composite cathode (5S–12KB) was significantly lower than that of the mechanically mixed sample (5S–12KB-MM), as shown in Fig. 4 . The reduced suspension viscosity may be related to the reduced porosity of the KB in the sulphur-impregnated KB slurry, compared with the untreated KB, due to the incorporation of sulphur particles. This effect is clearly demonstrated using suspensions with much higher sulphur content. We compare the rheological properties of 20.0 vol% sulphur–26.0 vol% KB composite (20S–26KB) suspension with a mechanically mixed suspension having 20.0 vol% sulphur–26.0 vol% KB (20S–26KB-MM). Interestingly, the sample obtained by mechanical mixing became a solid agglomerate ( Supplementary Fig. 3a ), whereas the S/C composite formed a smooth suspension ( Supplementary Fig. 3b ). In other words, the conventional mechanically mixed KB slurry with high concentration, larger than 13–26 vol%, is unable to form a colloidal solution and cannot flow. In contrast, the sulphur-impregnated KB slurry (20S–26KB) can form a uniform and flowable suspension at the same high KB and sulphur content ( Supplementary Fig. 3 ). The significantly reduced suspension viscosity associated with using S/C composite permits much higher allowable concentration of sulphur, which increases the theoretical capacity of the S/C catholyte. 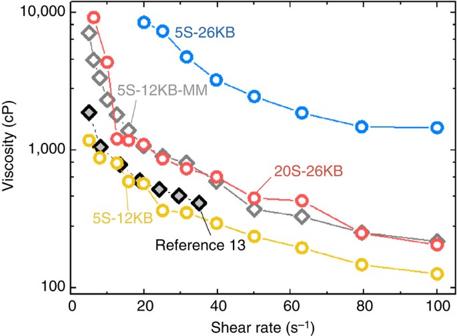Figure 4: Viscosity measurements of S/C catholytes. Viscosity versus shear rate of sulphur–carbon suspensions examined in this study in comparison with 22.4 vol% LiCoO2and 0.6 vol% KB in alkyl carbonate electrolyte reported by Dudutaet al.13Note that the 20S–26KB-MM sample formed a solid agglomerate (Supplementary Fig. 3a) and cannot be used for the viscosity test. Figure 4: Viscosity measurements of S/C catholytes. Viscosity versus shear rate of sulphur–carbon suspensions examined in this study in comparison with 22.4 vol% LiCoO 2 and 0.6 vol% KB in alkyl carbonate electrolyte reported by Duduta et al . [13] Note that the 20S–26KB-MM sample formed a solid agglomerate ( Supplementary Fig. 3a ) and cannot be used for the viscosity test. Full size image Influence of the concentration of carbon With the sulphur-impregnation approach, we increased the carbon content from 12 to 26 vol% while keeping the same sulphur content at 5 vol% (3.2 M [S]) to form the 5S–26KB catholyte. The first gravimetric discharge capacity of the 5S–26KB Li-suspension cell was higher than that of the 5S–12KB by ~20% ( Fig. 2 ). There is no significant change in the EIS response for the ohmic resistance and interfacial resistance between 5S–12KB and 5S–26KB Li-suspension cells ( Fig. 5a,b ). This suggests that further increase in the carbon content from 12 vol% to 26% leads to no improvement in the ohmic and interfacial resistance. Surprisingly, the charge-transfer resistance of the 5S–26KB Li-suspension cell is higher than that of the 5S–12KB sample ( Fig. 5c ). In addition, the viscosity of the 5S–26KB suspension is significantly larger than that of the 5S–12KB suspension by 5–10 times ( Fig. 4 ). We hypothesize that the increased charge-transfer resistance associated with high KB content results from the significantly increased suspension viscosity (~5–10-fold increase, Fig. 4 ). Further studies are on-going to understand the fundamental correlations between rheological and electrochemical properties of S/C composite catholytes. 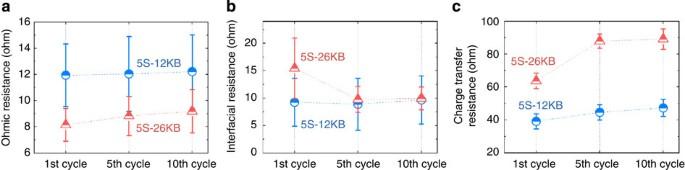Figure 5: EIS-fitting results of Li-suspension cells using 5S–12KB and 5S–26KB catholytes. (a) Ohmic resistance, (b) interfacial resistance and (c) charge-transfer resistance for 5S–12KB and 5S–26KB Li-suspension cells after 1st, 5th and 10th discharge/charge cycles. The EIS tests were replicated for three times. Figure 5: EIS-fitting results of Li-suspension cells using 5S–12KB and 5S–26KB catholytes. ( a ) Ohmic resistance, ( b ) interfacial resistance and ( c ) charge-transfer resistance for 5S–12KB and 5S–26KB Li-suspension cells after 1st, 5th and 10th discharge/charge cycles. The EIS tests were replicated for three times. Full size image Influence of the concentration of sulphur The concentration of sulphur determines the theoretical volumetric capacity of the catholyte, as discussed in Table 1 . We aim to maximize the volumetric concentration of sulphur without significantly increasing the viscosity of the catholyte. Here, we increased the concentration of sulphur from 5.0 vol% S (5S–26KB, 3.2 M [S]) to 20.0 vol% S (20S–26KB, 12.9 M [S]). Note that the concentration of KB (26 vol%) was chosen based on the minimum KB content inherently existing in the S/C composite (93.1 wt% sulphur and 6.9 wt% KB by thermogravimetric analysis, Supplementary Fig. 4 ) for a suspension having 20 vol% sulphur. The gravimetric discharge capacity of the 20S–26KB Li-suspension cell ( Fig. 2 , ~700 mAh g −1 ) was lower than that of the 5S–26KB sample ( Fig. 2 ~1,500 mAh g −1 ) by >50%, which can be attributed to the lower rate of utilization of sulphur associated with higher concentration of sulphur. However, the 20S–26KB catholyte delivered a twofold increase in volumetric capacity (286 Ah l −1 ) compared with the 5S–26 KB catholyte (128 Ah l −1 ). This demonstrates the advantage of employing catholyte with high sulphur concentration in achieving high volumetric capacity. The 20S–26KB suspension forms uniform and flowable catholyte ( Supplementary Fig. 3b ) with comparable viscosity to that of the semi-solid flow catholyte reported by Duduta et al . [13] (<1 vol% KB with mechanically mixed 22.4 vol% LiCoO 2 , Fig. 4 ). These observations support that the sulphur-impregnated slurry (20S–26KB) could work as a flowing catholyte. However, we note that the slurry property and flow ability will be gradually dictated more by the gravitational forces if KB and sulphur content are continuously increased. This is an important trade-off design consideration for the catholyte concept proposed in this study. Together, these observations highlight the unique advantage of using S/C composite catholyte, as it permits high concentration of active materials while it maintains proper viscosity in the suspension. Further optimization in increasing the concentration of sulphur and lowering the viscosity of the suspension may lead to further increase in the volumetric capacity and the electrochemical performance. Electrochemical and morphological reversibility To demonstrate the electrochemical reversibility of the S/C composite catholyte, we performed a cycling test of the 20S–26KB catholyte and examined the changes in the microstructure of the suspension via SEM at various discharge/charge stages. 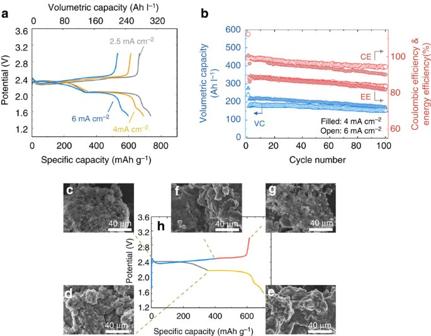Figure 6: Electrochemical performance and SEM images of 20S–26KB (12.9 M [S]) catholyte. (a) First galvanostatic discharge/charge profiles of Li-suspension cells using 20S–26KB S/C composite catholyte at 2.5, 4.0 (≡C/9) and 6.0 mA cm−2. (b) Cycling retention in the volumetric capacity (VC, based on catholyte), energy efficiency (EE) and coulombic efficiency (CE) of the 20S–26KB catholyte cells cycling at 4.0 (≡C/9) and 6.0 mA cm−2. (c–g) SEM images of the 20S–26KB catholyte at specified discharge/charge steps at 4 mA cm−2. (h) Representative discharge/charge profile of the 20S–26KB catholyte at 4 mA cm−2for illustration purpose. The electrochemical tests were replicated for more than three times. Figure 6a shows the first galvanostatic discharge/charge profile of the 20S–26KB Li-suspension cells at rates ranging from 2.5 to 6 mA cm −2 . Volumetric capacity ranging from 294 to 234 Ah l −1 was achieved based on the catholyte. To our knowledge, this system demonstrates one of the highest volumetric capacity of redox flow catholytes to date [12] , [23] , [24] . The superior volumetric capacity is resulted from the concentration of sulphur (20.0 vol% S or 12.9 M [S]) leading to high volumetric capacity 294–234 Ah l −1 . Figure 6b shows the cycling retention of the 20S–26KB catholyte at 4 and 6 mA cm −2 in volumetric capacity (left axis), coulombic efficiency (right axis) and energy efficiency (right axis). We note that the rates used in this work (2–6 mA cm −2 ) are comparable to other nonaqueous semi-solid flow-battery chemistries (2–10 mA cm −2 , Fig. 9 ) [12] , [23] , [24] , but significantly lower than the state-of-the-art aqueous flow-battery chemistries (for example, all-vanadium system 50–500 mA cm −2 , Fig. 9 ) [3] , [5] , [26] . Substantial decrease in volumetric capacity/efficiency only occurred after the first cycle, which could be attributed to the inefficiency of the lithium anode and/or the loss of polysulphide [44] . Since the 2 nd cycle ( Fig. 6b ), the cells achieved volumetric capacity retention of 79% (4 mA cm −2 ) and 85% (6 mA cm −2 ) after 100 cycles. In addition, high coulombic efficiency (90.3–94.5%) and energy efficiency (82–83.7%) after 100 cycles were achieved. The high volumetric capacity and electrochemical reversibility of the S/C catholyte suggest that the employment of the solid sulphur composite in catholyte is a promising direction for high-energy-density Li flow batteries. Figure 6: Electrochemical performance and SEM images of 20S–26KB (12.9 M [S]) catholyte. ( a ) First galvanostatic discharge/charge profiles of Li-suspension cells using 20S–26KB S/C composite catholyte at 2.5, 4.0 (≡C/9) and 6.0 mA cm −2 . ( b ) Cycling retention in the volumetric capacity (VC, based on catholyte), energy efficiency (EE) and coulombic efficiency (CE) of the 20S–26KB catholyte cells cycling at 4.0 (≡C/9) and 6.0 mA cm −2 . ( c – g ) SEM images of the 20S–26KB catholyte at specified discharge/charge steps at 4 mA cm −2 . ( h ) Representative discharge/charge profile of the 20S–26KB catholyte at 4 mA cm −2 for illustration purpose. The electrochemical tests were replicated for more than three times. Full size image Figure 9: Achieved catholyte volumetric capacity versus current density. Achieved catholyte volumetric capacities in this work (half-filled symbols) are compared with various reported work discussed earlier [12] , [23] , [24] . 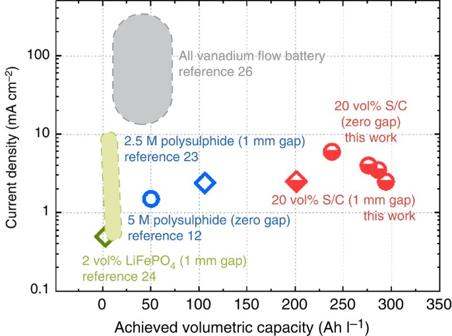Figure 9: Achieved catholyte volumetric capacity versus current density. Achieved catholyte volumetric capacities in this work (half-filled symbols) are compared with various reported work discussed earlier12,23,24. Open symbols were calculated from the work of Fanet al.23, Yanget al.12and Hamletet al.24The dotted green area denotes the range of the catholyte volumetric capacity (2.7–19 Ah l−1) achieved and current density used in the work of Hamletet al.24The dotted grey area denotes the state-of-the-art performance of all-vanadium flow batteries26. Open symbols were calculated from the work of Fan et al . [23] , Yang et al . [12] and Hamlet et al . [24] The dotted green area denotes the range of the catholyte volumetric capacity (2.7–19 Ah l −1 ) achieved and current density used in the work of Hamlet et al . [24] The dotted grey area denotes the state-of-the-art performance of all-vanadium flow batteries [26] . Full size image We exploited SEM to examine the changes in the microstructure at different stages of discharge/charge of the 20S–26KB Li-suspension cells, as shown in Fig. 6c–g . The SEM image of the pristine sample (before discharge, Fig. 6c ) shows submicron pores with uniform features. The S and C atoms are uniformly intermixed, as evidenced from the EDX mapping shown in Fig. 2 (20S–26KB). Upon discharge to the end of the first discharge plateau ( Fig. 6d ), large clusters (~10–15 μm) appeared with film-like deposits, which partially close the pores of the composite. The deposits may be related to precipitated polysulphides. This confirms that reduction of solid sulphur occurs directly on the carbon network in the suspension. Upon full discharge ( Fig. 6e ), the discharge product forms a continuous film that covers the entire composite and closes the pores. The film is attributed to Li–S solid discharge products such as Li 2 S (refs 28 , 30 , 44 , 45 ). An important open question arises as follows. Will the insulating discharge product/deposit/film be removed upon charging of the S/C suspension? (see further discussion in Fig. 7 ). Interestingly, upon charging to the first 50% of the capacity, small and scattered holes/pores/features reappeared ( Fig. 6f ), and finally, the porous features of the S/C composite recovered upon full recharge of the suspension ( Fig. 6g ). 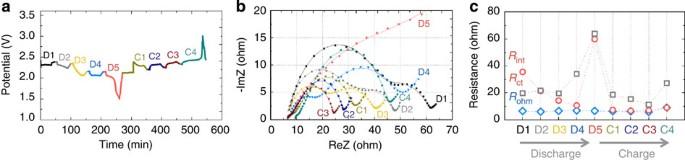Highly reversible morphological evolution of the catholyte highlights that the Li–S electrochemical reactions occur reversibly in the S/C composite network, having solid sulphur as the starting material and solid Li 2 S as the end products. Figure 7: Pseudo-in situEIS measurement. (a) Discharge and charge steps of the Li-suspension cells using 20S–26KB S/C composite catholyte. (b) EIS measurements during discharge (D1–D5, at open-circuit voltage (OCV)) and charge (C1–D4, at OCV). Each EIS measurement was measured after resting at OCV for 20 min. (c) The EIS-fitting results for the three resistance components (Rohm,RintandRct) during discharge/charge based on the equivalent circuit shown inFig. 3b. The pseudo-in situEIS tests were replicated for more than three times. Figure 7: Pseudo -in situ EIS measurement. ( a ) Discharge and charge steps of the Li-suspension cells using 20S–26KB S/C composite catholyte. ( b ) EIS measurements during discharge (D1–D5, at open-circuit voltage (OCV)) and charge (C1–D4, at OCV). Each EIS measurement was measured after resting at OCV for 20 min. ( c ) The EIS-fitting results for the three resistance components ( R ohm , R int and R ct ) during discharge/charge based on the equivalent circuit shown in Fig. 3b . The pseudo- in situ EIS tests were replicated for more than three times. Full size image To examine the reversibility of various impedance processes, we employed pseudo -in situ EIS measurement as the reaction proceeds. Figure 7a shows the discharge and charge steps of the 20S–26KB Li-suspension cells inserted with five EIS measurements ( Fig. 7b , D1–D5, at open-circuit voltage (OCV)) during discharge and four EIS measurements ( Fig. 7b , C1–C4, at OCV) during charging, as well as the fitting results of the three resistance components ( R ohm , R int and R ct ) [23] , [42] , [43] during discharge/charge ( Fig. 7c ). The ohmic resistance of the catholyte is the smallest among the three processes and is insensitive to the discharge/charge steps ( Fig. 7c ). The interfacial resistance first decreased upon discharge to polysulphide phases (D1–D4) and markedly increased upon full discharge (D5). This suggests that the interfacial resistance decreases by transforming the insulating solid sulphur to soluble polysulphides, which improves the interfacial contacts between sulphur-containing species and carbon [22] , but significantly increases due to the formation of insulating film-like Li 2 S (refs 28 , 30 , 44 , 45 ). Reversibly, the interfacial resistance decreased after charging the catholyte to the polysulphide phase (C1–C3) and remained small at the end of the charging. Finally, no significant increase in the charge-transfer resistance was noticed at the early stage of discharge (D1–D3, polysulphides) until the later stage of discharge (D4–D5), which is attributed to the formation of insulating Li 2 S solids, which blocks the charge transfer [42] , [46] . Reversibly, the charge-transfer resistance decreases upon charging of the catholyte, which is attributed to the formation of polysulphide species from decomposing the insulating Li 2 S solid. Overall, the SEM and pseudo -in situ EIS analysis reveal superior morphological reversibility and electrochemical reversibility of the S/C catholyte reported in this study. Flow cells under static and intermittent-flow modes We characterize the electrochemical performance of the S/C catholyte with a Li-flow cell configuration that adapts a 1.0-mm channel gap ( Fig. 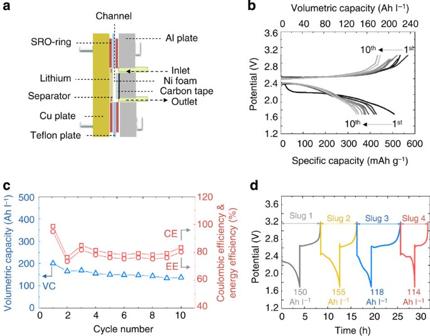8a ). Figure 8: Electrochemical performance in the 1-mm-channel-gap Li-flow cell. (a) Schematic illustration of the Li-flow cell configuration with a 1.0-mm-channel gap. (b) Galvanostatic discharge/charge cycle profiles (10 cycles) of the 20S–26KB catholyte in the Li-flow cell at a static mode at 2.5 mA cm−2. (c) Cycling retention in the volumetric capacity (VC, based on catholyte), energy efficiency (EE) and coulombic efficiency (CE) of the 20S–26KB catholyte in the Li-flow cell at a static mode at 2.5 mA cm−2. (d) Intermittent-flow tests of the 20S–26KB catholyte in the Li-flow cell at 4 mA cm−2. The flow channel dimensions are 1 × 2 × 10 mm. The electrochemical tests were replicated for more than three times. Figure 8b shows the discharge/charge cycling profiles of the 20S–26KB catholyte in the Li-flow cell under static condition. Catholyte volumetric capacity of 221 Ah l −1 was achieved with coulombic efficiency and energy efficiency >80% ( Fig. 8c ). We further performed an intermittent-flow test of the S/C catholyte, as the intermittent-flow mode was suggested to be a more effective operation mode for the semi-solid flow battery [13] . Figure 8d shows four iterations of charge/discharge profiles of the 20S–26KB catholyte in an intermittent-flow mode at 4 mA cm −2 , demonstrating catholyte volumetric capacity between 110–155 Ah l −1 . The power output of the semi-solid sulphur flow cell is comparable to other nonaqueous semi-solid flow cells [13] , [24] , but significantly lower than aqueous flow cells [3] , [5] , [26] . Further improvements on the single-cell stack design, electrical conductivity and interfacial contacts in the flow cathode are expected to improve the power output of the semi-solid sulphur flow system. Figure 8: Electrochemical performance in the 1-mm-channel-gap Li-flow cell. ( a ) Schematic illustration of the Li-flow cell configuration with a 1.0-mm-channel gap. ( b ) Galvanostatic discharge/charge cycle profiles (10 cycles) of the 20S–26KB catholyte in the Li-flow cell at a static mode at 2.5 mA cm −2 . ( c ) Cycling retention in the volumetric capacity (VC, based on catholyte), energy efficiency (EE) and coulombic efficiency (CE) of the 20S–26KB catholyte in the Li-flow cell at a static mode at 2.5 mA cm −2 . ( d ) Intermittent-flow tests of the 20S–26KB catholyte in the Li-flow cell at 4 mA cm −2 . The flow channel dimensions are 1 × 2 × 10 mm. The electrochemical tests were replicated for more than three times. Full size image We demonstrate a new flow cathode that employs a highly concentrated sulphur-impregnated carbon composite, and show high catholyte volumetric capacity (294–192 Ah l −1 ) with long cycle life (>100 cycles), high columbic efficiency (90–94.5% at 100th cycle) and energy efficiency (82–83.7% at 100th cycle). Pseudo -in situ EIS and SEM techniques revealed superior electrochemical and morphological reversibility of the S/C catholyte. Figure 9 shows the achieved catholyte volumetric capacity reported in this work (both in ‘zero-gap’ and ‘1-mm-gap’ cells) in comparison with reported Li-flow-cathode chemistries at various current densities [12] , [23] , [24] . The highly concentrated (20 vol% S, 12.9 M [S]) sulphur-impregnated carbon composite catholyte introduced in this work demonstrates substantial improvement in volumetric capacity compared with other aqueous [3] , [5] , [26] and nonaqueous [12] , [23] , [24] flow chemistries ( Fig. 9 ). In addition, the solid-sulphur flow cathode exhibits similar power capability compared with other nonaqueous semi-solid flow chemistries [13] , [24] , but significantly lower power output compared with the aqueous all-vanadium flow batteries [3] , [5] , [26] . The hybrid configuration used in our study limits the scalability of the negative electrode [17] , which can be improved by replacing the lithium metal with semi-solid negative flow catholytes such as the semi-solid silicon anolyte [27] . Our concept of impregnating insulating solid active materials with a conductive carbon network offers a promising direction to further increase the energy density and cycling reversibility of RFBs and semi-solid flow batteries. Materials All chemicals were used as received. Ketjen Black EC-600JD (KB) was received from AzkoNobel. Sulphur, lithium nitrate (LiNO 3 ), lithium perchlorate (LiClO 4 ), 1,3-dioxolane (DOL) and 1,2-dimethoxyethane(DME) were received from Sigma-Aldrich. Carbon paper (HCP010N) was received from Shanghai Hesen Electric Co. Ltd. Lithium foil was received from Shenzhen Meisen Electromechanical Co. Ltd.). Preparation of the S/C composite The S/C composite was prepared according to the well-established method for traditional solid sulphur electrodes [28] , [29] , [30] , [31] , [32] , [33] , [34] , [35] , [36] , [37] , [38] . Sulphur and KB were mixed with a mass ratio 22:1 in DME, followed by sonication using the SLPt Cell Disruptor (Branson, USA) for 30 min. The sulphur and KB mixture was first air dried at 25 °C for 2 h to remove most of the solvent followed by heat treatment at 155 °C for 6 h for sulphur impregnation. The chemical composition of the S/C composite was determined to be 93.1 wt.% sulphur and 6.9 wt.% KB by thermogravimetric analysis, Supplementary Fig. 4 . Preparation of the S/C suspension All the suspensions reported herein were made with an electrolyte of 0.2 M LiClO 4 and 0.1 M LiNO 3 in DOL and DME (volume ratio 1:1). The active materials (sulphur or S/C composite) and KB were mixed in a 10-ml glass container with the electrolyte, followed by sonication using the SLPt Cell Disruptor for 10 min before testing. Assembly of the Li-suspension cell or zero-gap cell Supplementary Fig. 1 shows the structure of the Li-suspension cell or ‘zero-gap’ cell. One piece of lithium foil (20 mm diameter) was placed onto the bottom stainless steel cell body. Two Celgard 2325 separators (25 mm diameter) were placed on the lithium foil. Electrolyte (100 μl) (0.2 M LiClO 4 and 0.1 M LiNO 3 in DOL and DME (1:1 v/v)) was added on the separators. One piece of carbon paper (18 mm diameter) was placed on the separator act as a buffer layer to decrease the shuttle effect and enhance the conductivity, as suggested by the work of Manthiram et al . [47] , [48] Ten μl suspension was added on the surface of the carbon paper. A piece of nickel foam (18 mm diameter) was placed on the suspension as a current collector followed by a stainless steel spring and a polytetrafluoroethylene O-ring. The effective geometric surface area of the suspension was smaller than the carbon interlayer and current collector and was measured to be 0.2 cm 2 . Two cell bodies (bottom and top) were separated by a polytetrafluoroethylene spacer to avoid a short circuit. The cell assembly process was conducted in an Ar-filled glove box (Etelux, <0.1 p.p.m. of H 2 O and <0.1 p.p.m. O 2 ). Assembly of the Li-flow cell or 1-mm-gap cell Figure 8a shows the structure of the Li-flow cell or ‘1-mm-gap’ cell. One piece of lithium foil (2 × 10 mm) was attached to a copper (Cu) cell body, which acted as a current collector for the negative electrode. Two Celgard 2325 separators (4 × 14 mm) were placed on the surface of the lithium foil followed by adding 50 μl of electrolyte. A teflon channel spacer (1 mm thickness) was placed between the copper cell body and a piece of pressed nickel foam was attached to an outer aluminium (Al) cell body as a current collector fixed by six bolts. Twenty μl catholytes were injected into the channel (1 × 2 × 10 mm) from the Al plate inlet by a SPLab02 syringe pump (Baoding Shenchen Precision Pump Co. Ltd., China). The Li-flow cell assembly process was conducted in an Ar-filled glove box (Etelux, <0.1 p.p.m. of H 2 O and <0.1 p.p.m. O 2 ). Electrochemical characterizations All the electrochemical characterizations were performed using a VMP3 electrochemical testing unit (Bio-Logic). Galvanostatic charge/discharge tests were performed between 1.5 and 3.0 V versus Li + /Li. Current density was calculated based on the effective geometric surface area of the catholyte in the ‘zero-gap’ cell (0.2 cm 2 ) and ‘1-mm-gap’ cell (0.2 cm 2 ). The specific capacity was calculated from the mass of active materials of sulphur. The volumetric capacity was calculated from the total volume of the suspension. The energy density was calculated by integrating the discharge capacity and voltage normalized by the total volume of the suspension. EIS measurements used sinusoidal voltage oscillations of 20 mV amplitude at the OCV of the cells. The oscillation frequencies were swept from 100 kHz to 100 mHz with three repetitions for every test. An equivalent circuit shown in Fig. 3b was used to fit all the EIS data by a nonlinear calculation method [23] , [42] , [43] . Material characterizations SEM characterization was performed on Quanta 400 FEI. The SEM samples for different discharge/charge steps ( Fig. 6c–g ) were collected from cells disassembled at specified discharge/charge steps ( Fig. 6c–g ) in the glove box. The residual solvent was evaporated before SEM observing. The viscometric behaviours of various suspensions were measured using Physica MCR 301, Anton Paar. The viscosity was recorded as a function of the shear rate (increasing) and obtained from the RHEOPLUS software. How to cite this article : Chen, H. et al . Sulphur-impregnated flow cathode to enable high-energy-density lithium flow batteries. Nat. Commun. 6:5877 doi: 10.1038/ncomms6877 (2015).